Cardiac arrhythmia induced by genetic silencing of ‘funny’ (f) channels is rescued byGIRK4inactivation The mechanisms underlying cardiac automaticity are still incompletely understood and controversial. Here we report the complete conditional and time-controlled silencing of the ‘funny’ current ( I f ) by expression of a dominant-negative, non-conductive HCN4-channel subunit (hHCN4-AYA). Heart-specific I f silencing caused altered [Ca 2+ ] i release and Ca 2+ handling in the sinoatrial node, impaired pacemaker activity and symptoms reminiscent of severe human disease of pacemaking. The effects of I f silencing critically depended on the activity of the autonomic nervous system. We were able to rescue the failure of impulse generation and conduction by additional genetic deletion of cardiac muscarinic G-protein-activated (GIRK4) channels in I f -deficient mice without impairing heartbeat regulation. Our study establishes the role of f -channels in cardiac automaticity and indicates that arrhythmia related to HCN loss-of-function may be managed by pharmacological or genetic inhibition of GIRK4 channels, thus offering a new therapeutic strategy for the treatment of heart rhythm diseases. Heart automaticity is a fundamental physiological function in animals. Pacemaker activity is generated by specialized, spontaneously active myocytes localized to the sinoatrial node (SAN). The SAN with its fastest spontaneous beating rate generates the cardiac impulse and controls the heartbeat. In the case of SAN failure, other components of the conduction system such as the atrioventricular node (AVN) and the His-Purkinje fibre (PF) network can also generate viable pacemaking [1] . Dysfunction in SAN automaticity underlies congenital or acquired bradycardia and bradycardia-associated conditions. Furthermore, it contributes to debilitating symptoms such as syncope, atrial fibrillation and heart failure, and causes sudden death [2] , [3] , [4] , [5] . SAN disease and conduction block account for more than 450,000 electronic pacemaker implantations each year in Europe and North America [6] . Thus, there is a strong interest in elucidating the mechanisms underlying cardiac pacemaking and impulse conduction at both the fundamental and clinical levels, and in finding alternative treatment options. The ability of SAN cells to generate the pacemaker action potential is due to the diastolic depolarization phase during which the membrane voltage, from the end of an action potential, slowly depolarizes to reach the firing threshold for the succeeding one. The slope of the diastolic depolarization continuously modulates the heart rate (HR) and is regulated in opposite directions by the sympathetic and parasympathetic branches of the autonomic nervous system. Different classes of membrane ion channels, as well as ryanodine receptors of the sarcoplasmic reticulum, are involved in the generation and regulation of the diastolic depolarization (see ref. 1 for review), but their specific functional roles are still incompletely understood. Among cardiac ion channels, f - (HCN) channels, underlying the hyperpolarization-activated I f current, are thought to play a major role in the generation and autonomic regulation of the diastolic depolarization in the SAN and in the cardiac conduction system [7] , [8] , but its functional role is still a matter of controversy [9] . A family of four homologous HCN-channel subunit isoforms (HCN1–4) was identified in mammals [10] , [11] , [12] , [13] . HCN4 is the predominant f -channel isoform in the mouse SAN and in the conduction system [14] . HCN1 and HCN2 are also present in the conduction system at varying expression levels [14] , [15] . Recent studies have indicated that human HCN4-channel mutations underlie congenital alterations in SAN pacemaking in humans, with variable symptoms ranging from mild or moderate bradycardia [16] , [17] , [18] to chronotropic incompetence [19] , or atrioventricular conduction block with ventricular tachycardia [20] . HCN4 knockout mice show a reduction of ~70% in I f current associated with varying degrees of dysfunction in heart automaticity, ranging from recurrent SAN pauses with no significant change in HR and autonomic responsiveness [21] , [22] to lethal ventricular bradycardia and heart block [23] . These discrepancies could be explained by the different strategies of gene targeting adopted and/or by the presence of the other HCN-channel isoforms that can compensate for the loss-of-function of HCN4 channels in both the SAN and cardiac conduction system. Furthermore, deletion of the HCN4 protein may lead to alterations in the function of channel-associated proteins. We thus developed a conditional transgenic mouse model expressing non-conducting hHCN4 subunits to suppress I f conductance, independent of the endogenously expressed HCN subunits, to study the importance of this current in the generation and conduction of the cardiac impulse. We show that complete silencing of I f alters intracellular Ca 2+ handling in pacemaker myocytes and thus causes a complex disorder of cardiac rhythm, including SAN failure, atrioventricular block (AVB) and ventricular arrhythmia, which could be prevented by genetic inactivation of G-protein-activated (GIRK4) channels. In summary, our study provides a new animal model of human pathologies of HR and rhythm, and identifies a new potential pharmacological target for the treatment of bradycardia. Generation of conditional hHCN4-AYA-expressing transgenic mice To suppress I f conductance in a cardiac-specific and time-controlled manner, we generated double-transgenic mutant (Mut) mice expressing hHCN4-AYA dominant-negative subunits and a tetracycline-sensitive transactivator (tTA [24] ) under the control of an α-myosin heavy chain (αMHC) promoter [25] . In the absence of doxycycline (DOX), tTA binds to its promoter and drives the expression of an hHCN4 pore mutant construct in which a haemagglutinin (HA) epitope tag was added to the amino terminus and the selectivity filter motif was mutated to hHCN4-G480A/G482A (hHCN4-AYA; Fig. 1a ). Two-electrode voltage-clamp recordings in Xenopus oocytes after coexpression of hHCN4-AYA cRNA with wild-type mHCN4 or mHCN2 cRNAs showed that mutated hHCN4-AYA protein affected mHCN2 and mHCN4 subunit-mediated currents in a dominant-negative manner ( Supplementary Fig. 1a ). 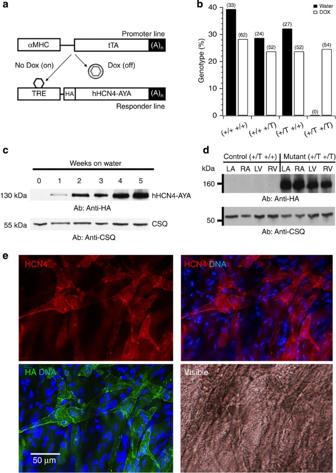Figure 1: Generation of transgenic mutant mice. (a). Schematic illustration of the Tet-off system: The tetracycline-dependent transactivator (tTA) is expressed under the control of the αMHC promoter. In the heart of double-transgenic (mutant) animals, tTA binds to the tetracycline-responsive element (TRE), resulting in the expression of HA-hHCN4-AYA (hHCN4-AYA). A conformational change of tTA after the binding of DOX inhibits transgene expression. (b) Percentage of genotypes obtained after breeding of the promoter line (first locus) and responder line (second locus) on water (black bars) or DOX (white bars). Absolute animal numbers are given in parentheses above the bars. (c) Detection of transgenic hHCN4-AYA protein after 0 to 5 weeks after DOX withdrawal by western blotting. Total heart lysates were analysed with antibodies against the HA-Tag and calsequestrin (CSQ). (d) Western blotting analysis of protein isolated from the left atrium (LA), right atrium (RA), left ventricle (LV) and right ventricle (RV) of control and mutant mice. Different tissues lysates were analysed with antibodies against the HA-Tag and CSQ. (e) Cellular expression of hHCN4-AYA protein in (n=4) SAN preparations (seeSupplementary Fig. 2) isolated from mutant mice. Expression was evaluated by using anti-HCN4 (red, top-left panel) and anti-HA (green, bottom-left panel) antibodies. Staining of nuclei is shown in blue (top-right and bottom-left panels). Bottom-right panel: bright-field image of tissue. Scale bar, 50 μm. Figure 1: Generation of transgenic mutant mice. ( a ). Schematic illustration of the Tet-off system: The tetracycline-dependent transactivator (tTA) is expressed under the control of the αMHC promoter. In the heart of double-transgenic (mutant) animals, tTA binds to the tetracycline-responsive element (TRE), resulting in the expression of HA-hHCN4-AYA (hHCN4-AYA). A conformational change of tTA after the binding of DOX inhibits transgene expression. ( b ) Percentage of genotypes obtained after breeding of the promoter line (first locus) and responder line (second locus) on water (black bars) or DOX (white bars). Absolute animal numbers are given in parentheses above the bars. ( c ) Detection of transgenic hHCN4-AYA protein after 0 to 5 weeks after DOX withdrawal by western blotting. Total heart lysates were analysed with antibodies against the HA-Tag and calsequestrin (CSQ). ( d ) Western blotting analysis of protein isolated from the left atrium (LA), right atrium (RA), left ventricle (LV) and right ventricle (RV) of control and mutant mice. Different tissues lysates were analysed with antibodies against the HA-Tag and CSQ. ( e ) Cellular expression of hHCN4-AYA protein in ( n =4) SAN preparations (see Supplementary Fig. 2 ) isolated from mutant mice. Expression was evaluated by using anti-HCN4 (red, top-left panel) and anti-HA (green, bottom-left panel) antibodies. Staining of nuclei is shown in blue (top-right and bottom-left panels). Bottom-right panel: bright-field image of tissue. Scale bar, 50 μm. Full size image Heart-specific expression of hHCN4-AYA during pregnancy resulted in embryonic lethality, which is similar to that described in homozygous HCN4 −/− mice [26] , because no double-transgenic mutant mice were born (+/T +/T, Fig. 1b . The likelihood of the other possible genotypes was ~30% ( n (+/+ +/+)=33, n (+/+ +/T)=24 and n (+/T +/+)=27). When hHCN4-AYA expression was suppressed by administering DOX to the mothers during pregnancy, the animals were born at a normal Mendelian ratio ( n (+/+ +/+)=62, n (+/+ +/T)=52, n (+/T +/+)=52 and n (+/T +/T)=54). DOX withdrawal at weaning induced expression of hHCN4-AYA, which was detectable after 1 week ( Fig. 1c and Supplementary Fig. 1b ). The expression level increased and resulted in a stronger protein signal after 2–3 weeks, reaching a maximum level after 4 weeks. The mutant hHCN4-AYA protein was detected in all cardiac chambers, with the highest expression in the atria ( Fig. 1d and Supplementary Fig. 1b ). To verify that the αMHC promoter effectively induced expression of hHCN4-AYA protein in pacemaker myocytes, we studied anti-HCN4 and anti-HA immunoreactivities by macro-confocal microscopy in preparations of the whole supraventricular stage of the heart containing the SAN and AVN of control ( Supplementary Fig. 2 ) and mutant mice ( Supplementary Fig. 3 ). Individual cells in the intact mutant SAN showed strong membrane-bound anti-HA immunoreactivity consistent with hHCN4-AYA protein expression ( Fig. 1e ). SAN–AVN preparations of the mutant heart displayed expression of hHCN4-AYA protein in all identifiable myocytes of the two heart pacemaker centres ( Fig. 2 ). Inside the SAN region, the density of hCN4-AYA-expressing cells was particularly high in the site of origin of the pacemaker activity described in previous studies [27] , [28] . Similar to that in SAN, hHCN4-AYA-expressing cells were densely distributed throughout the whole AVN region ( Fig. 2 and Supplementary Fig. 3 ). No anti-HA immunoreactivity was found in preparations obtained from control mice ( Supplementary Fig. 4 ). A significant population of hHCN4-AYA-expressing cells in the SAN and AVN stained positively against anti-HCN1 immunoreactivity ( Fig. 2 ), which was also expressed in pacemaker cells of the SAN and AVN [14] . In addition, we performed immunostaining of enzymatically isolated SAN and AVN myocytes of control and mutant mice [29] . All myocytes isolated from mutant mice showed strong plasma membrane anti-HA immunoreactivity ( Supplementary Fig. 5 ). 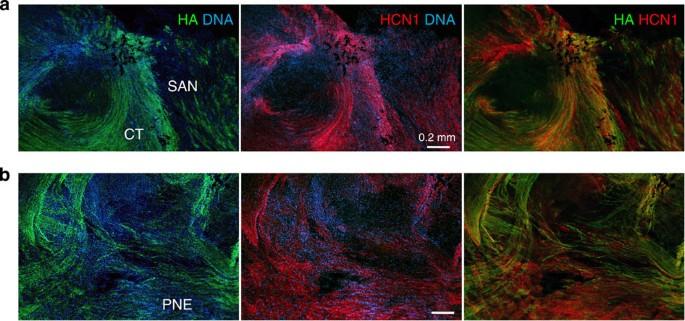Figure 2: Transgene expression in the SAN and AVN regions of heart nodal tissues. Representative whole-mount stainings ofn=4 mouse heart nodal tissues with close-up views of the mutant SAN (a) and AVN (b) regions stained with anti-HA (green) and anti-HCN1 (red) antibodies. Stainings of nuclei are shown in blue. SeeSupplementary Fig. 3for the localization of the close-up views in whole-mount right atrial preparations containing the nodes. Scale bar, 200 μm. Figure 2: Transgene expression in the SAN and AVN regions of heart nodal tissues. Representative whole-mount stainings of n =4 mouse heart nodal tissues with close-up views of the mutant SAN ( a ) and AVN ( b ) regions stained with anti-HA (green) and anti-HCN1 (red) antibodies. Stainings of nuclei are shown in blue. See Supplementary Fig. 3 for the localization of the close-up views in whole-mount right atrial preparations containing the nodes. Scale bar, 200 μm. Full size image Expression of hHCN4-AYA in mutant mice silenced I f conductance in SAN and conduction system To evaluate the functional effects of hHCN4-AYA expression on I f in the SAN and in the cardiac conduction system, we recorded I f in control and mutant mice deprived of DOX after weaning. To unambiguously quantify current densities, we defined I f as the net Ba 2+ -insensitive and Cs + -sensitive current [29] , [30] ( Fig. 3 ). To record I f in PF myocytes, we crossed control and mutant mice with Cx40 +/EGFP mice (Mut/ Cx40 +/EGFP , see Methods) [31] . In Mut/ Cx40 +/EGFP mice, PF myocytes were identified by enhanced green fluorescent protein (EGFP) epifluorescence. In comparison with controls, the averaged cellular capacitance was increased in mutant myocytes, indicating an increase in cell size in the conduction system of mutant mice ( Supplementary Fig. 6 ). In myocytes isolated from control mice, the density of I f was highest in SAN and lower in AVN and PF myocytes, as reported previously [32] . Unlike in control myocytes, I f was drastically reduced at all membrane voltages tested in SAN, AVN and PF myocytes isolated from mutant mice. We did not detect I f at voltages spanning the diastolic depolarization range in all mutant myocytes tested (−75/−35 mV, Fig. 3 ). 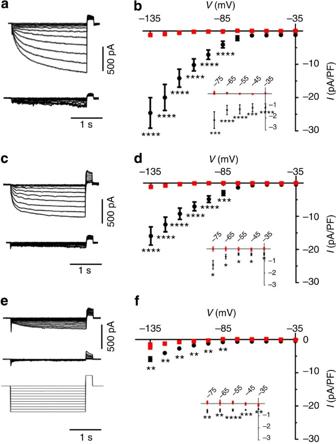Figure 3:Ifin control and mutant pacemaker myocytes. Representative examples ofIfrecordings (Cs+-sensitive current, (a)) averaged current-to-voltage (I/V) curve (b) in control (n=11) and mutant (n=14) SAN pacemakers myocytes; (c,d)Ifrecordings andI/Vcurve in AVN myocytes from control (n=16) and mutant (n=10) mice. (e,f)Ifrecordings andI/Vcurve in myocytes from control (n=12) and mutant (n=9) PF myocytes. In (a,b,e) the top panel showsIfin control myocytes and the bottom panel showsIfin mutant myocytes. Inb,d,f, black circles indicate control and red squares indicate mutant myocytes. Statistical significance was tested at each voltage using the unpairedt-test. *P<0.05, **P<0.01, ***P<0.001, ****P<0.0001. Error bars indicate s.e.m. The voltage-clamp protocol used for all the recordings is shown ine. Figure 3: I f in control and mutant pacemaker myocytes. Representative examples of I f recordings (Cs + -sensitive current, ( a )) averaged current-to-voltage ( I / V ) curve ( b ) in control ( n =11) and mutant ( n =14) SAN pacemakers myocytes; ( c , d ) I f recordings and I / V curve in AVN myocytes from control ( n =16) and mutant ( n =10) mice. ( e , f ) I f recordings and I / V curve in myocytes from control ( n =12) and mutant ( n =9) PF myocytes. In ( a , b , e ) the top panel shows I f in control myocytes and the bottom panel shows I f in mutant myocytes. In b , d , f , black circles indicate control and red squares indicate mutant myocytes. Statistical significance was tested at each voltage using the unpaired t -test. * P <0.05, ** P <0.01, *** P <0.001, **** P <0.0001. Error bars indicate s.e.m. The voltage-clamp protocol used for all the recordings is shown in e . Full size image I f silencing slowed basal pacemaker activity and induced delayed afterdepolarization in SAN, AVN and PF myocytes Mutant SAN myocytes had significantly lower spontaneous firing rates than control myocytes and showed a strong reduction in the diastolic depolarization slope, both during the linear and exponential phases, as well as in the upstroke velocity ( Supplementary Table 1 ). β-Adrenergic receptor stimulation with submaximal (2 nM) or maximal (100 nM) concentrations of isoproterenol (ISO) increased the spontaneous beating rate in both control and mutant cells in a concentration-dependent manner. The difference in rate between mutant and control myocytes was present at all ISO concentrations tested ( Fig. 4a,b ). Analysis of the action potential properties of mutant SAN myocytes under basal non-stimulated conditions revealed a more negative action potential threshold, prolonged action potential duration and reduced action potential amplitude. Control and mutant SAN myocytes showed spontaneous diastolic depolarizations of the membrane potential (delayed afterdepolarizations, DADs) that did not elicit an action potential ( Fig. 4a,c ). Under basal conditions (no ISO), the frequency of DADs was significantly higher in mutant than in control myocytes ( Fig. 4c ). ISO significantly reduced the frequency of DADs in control but not in mutant myocytes ( Fig. 4c ). As a consequence, the frequency of DADs in mutant cells under ISO was more than tenfold higher than that recorded in control myocytes. The diastolic interval between a DAD and the following action potential under ISO was significantly longer than the cycle length between the two consecutive action potentials preceding the DAD ( Fig. 4d ), suggesting that DADs delayed the formation of the following pacemaker impulse. Similar results were obtained in mutant AVN and PF myocytes under basal conditions or ISO ( Fig. 4e–l ). DADs were consistently recorded also in AVN and PF myocytes and displayed properties similar to those seen in SAN cells. Apart from longer action potential durations in mutant AVN cells, no differences were found in action potential parameters between mutant and control AVN and PF myocytes at baseline ( Supplementary Table 1 ). The very low basal pacemaker activity recorded in mutant PF myocytes was also increased by ISO application, but—similar to our findings in SAN and AVN—the difference in spontaneous beating rates between control and mutant cells remained ( Fig. 4e,f ). Taken together, our data show that I f is critical for setting the basal spontaneous beating rate in SAN, AVN and PF myocytes, but is not required for the sympathetic regulation of pacemaking in these structures. In addition, I f silencing favoured the induction of DADs in spontaneously beating myocytes. 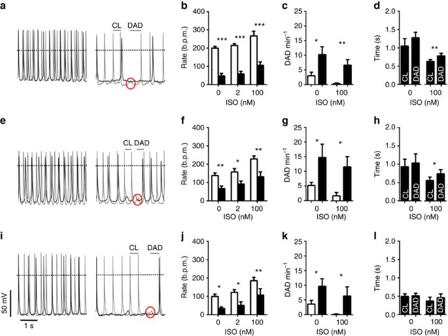Figure 4: Pacemaker activity and DADs in control and mutant myocytes. (a) Action potential recordings of control (left) or mutant (right) SAN myocytes in Tyrode’s solution (black line) and ISO (100 nM, grey line). (b) Averaged spontaneous beating rates of SAN myocytes in Tyrode’s solution (0;n=11 control,n=11 mutant), ISO 2 nM (n=10 control,n=11 mutant) or 100 nM (n=7 control,n=10 mutant) expressed in beats min−1(b.p.m.). (c) Frequency of DADs (defined as a variation of at least 5 mV of the membrane potential) in control and mutant SAN myocytes in Tyrode’s solution (n=10 control,n=14 mutant) or ISO 100 nM (n=10 control,n=12 mutant). (d) Averaged time interval between a DAD and the following action potential (DAD) in comparison with the cycle length (CL) of the two consecutive action potentials preceding the DAD inn=8 mutant SAN myocytes. (e) Action potentials of control (left) or mutant (right) AVN myocytes in Tyrode’s solution (black line) and after ISO (100 nM) perfusion (gray line). (f) Spontaneous rates of AVN myocytes in Tyrode’s and ISO (0:n=12 control,n=9 mutant cells; 2:n=9 control,n=7 mutant; 100:n=6 control,n=7 mutant). (g) Frequency of DADs in control and mutant AVN myocytes in Tyrode’s and ISO (0:n=11 control,n=11 mutant; 100:n=11 control,n=13 mutant). (h) Same data as indfor AVN mutant myocytes (0,n=9) and in ISO (100,n=6). (i) Spontaneous action potentials recorded from PF myocytes from control (left) or mutant (right) mice in Tyrode’s solution (black line) and after perfusion of ISO (100 nM, grey line). (j) Spontaneous beating rates of PF myocytes (0:n=10 control,n=7 mutant; 2:n=9 control,n=6 mutant; 100:n=7 control,n=5 mutant). (k) Frequency of DADs in control and mutant PF myocytes (0:n=10 control andn=8 mutant; 100:n=5 control,n=7 mutant). (l) Same data as indandhfor PF mutant myocytes in Tyrode’s solution (n=6) and ISO (n=3) in mutant PF myocytes. Statistics: two-way analysis of variance followed by Sidak multiple comparisons test and unpaired or pairedt-test. *P<0.05, **P<0.01, ***P<0.001. Error bars indicate s.e.m. Dotted line indicates the 0 mV. Open bars represent data from control, filled bars from mutant mice. Figure 4: Pacemaker activity and DADs in control and mutant myocytes. ( a ) Action potential recordings of control (left) or mutant (right) SAN myocytes in Tyrode’s solution (black line) and ISO (100 nM, grey line). ( b ) Averaged spontaneous beating rates of SAN myocytes in Tyrode’s solution (0; n =11 control, n =11 mutant), ISO 2 nM ( n =10 control, n =11 mutant) or 100 nM ( n =7 control, n =10 mutant) expressed in beats min − 1 (b.p.m.). ( c ) Frequency of DADs (defined as a variation of at least 5 mV of the membrane potential) in control and mutant SAN myocytes in Tyrode’s solution ( n =10 control, n =14 mutant) or ISO 100 nM ( n =10 control, n =12 mutant). ( d ) Averaged time interval between a DAD and the following action potential (DAD) in comparison with the cycle length (CL) of the two consecutive action potentials preceding the DAD in n =8 mutant SAN myocytes. ( e ) Action potentials of control (left) or mutant (right) AVN myocytes in Tyrode’s solution (black line) and after ISO (100 nM) perfusion (gray line). ( f ) Spontaneous rates of AVN myocytes in Tyrode’s and ISO (0: n =12 control, n =9 mutant cells; 2: n =9 control, n =7 mutant; 100: n =6 control, n =7 mutant). ( g ) Frequency of DADs in control and mutant AVN myocytes in Tyrode’s and ISO (0: n =11 control, n =11 mutant; 100: n =11 control, n =13 mutant). ( h ) Same data as in d for AVN mutant myocytes (0, n =9) and in ISO (100, n =6). ( i ) Spontaneous action potentials recorded from PF myocytes from control (left) or mutant (right) mice in Tyrode’s solution (black line) and after perfusion of ISO (100 nM, grey line). ( j ) Spontaneous beating rates of PF myocytes (0: n =10 control, n =7 mutant; 2: n =9 control, n =6 mutant; 100: n =7 control, n =5 mutant). ( k ) Frequency of DADs in control and mutant PF myocytes (0: n =10 control and n =8 mutant; 100: n =5 control, n =7 mutant). ( l ) Same data as in d and h for PF mutant myocytes in Tyrode’s solution ( n =6) and ISO ( n =3) in mutant PF myocytes. Statistics: two-way analysis of variance followed by Sidak multiple comparisons test and unpaired or paired t -test. * P <0.05, ** P <0.01, *** P <0.001. Error bars indicate s.e.m. Dotted line indicates the 0 mV. Open bars represent data from control, filled bars from mutant mice. Full size image I f silencing induced augmented SR Ca 2+ load and an increased frequency of local Ca 2+ release events in SAN myocytes The high frequency of DAD occurrence in I f -deficient mutant myocytes isolated from the three rhythmogenic centres suggested altered Ca 2+ handling and release in these cells [33] . We therefore recorded in control and mutant SAN cells voltage-dependent Ca 2+ currents using voltage-clamp experiments and intracellular Ca 2+ release ([Ca 2+ ] i ) by line-scan imaging of Fluo-4-loaded myocytes ( Fig. 5 ). Quantification of voltage-dependent Ca 2+ currents revealed an increased density of I Ca,L , while the density and activation of I Ca,T were unchanged ( Supplementary Fig.7 ). Consistent with our current clamp recordings ( Fig. 4 ), the frequency of spontaneous [Ca 2+ ] i transients was reduced in mutant SAN cells ( Fig. 5a ). Under basal conditions, mutant cells showed a significantly higher frequency of local Ca 2+ release events (LCRs, Fig. 5b ) and increased amplitude of [Ca 2+ ] i transients ( Fig. 5c ), indicating augmented sarcoplasmic reticulum (SR) Ca 2+ load in these myocytes. Perfusion with ISO (100 nM) reduced the frequency of LCRs, but increased the frequency and reduced the amplitude of [Ca 2+ ] i transients ( Fig. 5d ) in mutant SAN cells. We did not observe differences in the upstroke velocity, duration or recovery time of spontaneous [Ca 2+ ] i transients ( Supplementary Fig. 8 ). We then directly tested the status of the SR Ca 2+ load in isolated control and mutant SAN myocytes under ISO by rapid caffeine (10 mM) application. Caffeine-evoked Ca 2+ release was significantly higher in mutant than in control cells, but the decay of Ca 2+ release was similar in myocytes from the two mouse strains ( Fig. 5e ). As it is known that SR Ca 2+ overload favours the formation of [Ca 2+ ] i waves leading to Na + /Ca 2+ exchanger activation-mediated DADs in cardiomyocytes [34] , we quantified the frequency of [Ca 2+ ] i waves ( Fig. 5f,g ). Under basal conditions and ISO, the frequency of [Ca 2+ ] i waves in mutant SAN myocytes ( Fig. 5h,i ) was comparable to the frequency of DADs ( Fig. 4c ). Under ISO, the diastolic interval between a [Ca 2+ ] i wave and the following spontaneous [Ca 2+ ] i transient was significantly longer than the cycle length between the two consecutive spontaneous [Ca 2+ ] i transients preceding the [Ca 2+ ] i wave ( Fig. 5k ). This observation is consistent with the hypothesis that [Ca 2+ ] i waves induced DADs in mutant myocytes. 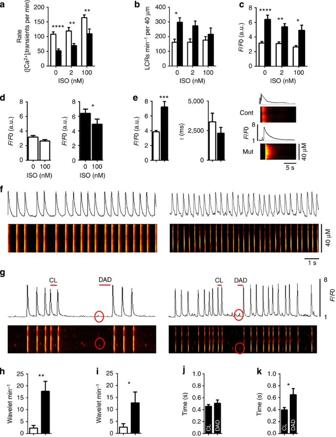Figure 5: [Ca2+]ihandling inIf–deficient SAN myocytes. (a) Averaged frequency of spontaneous [Ca2+]itransients of SAN myocytes in Tyrode’s solution (n=20 control,n=29 mutant cells), ISO 2 nM (n=16 control,n=29 mutant cells) and in ISO 100 nM (n=14 control,n=12 mutant cells). (b) Frequency of LCRs in Tyrode-perfused SAN myocytes (n=19 control,n=24 mutant cells), in ISO 2 nM (n=18 control andn=26 mutant cells) and ISO 100 nM (n=14 control,n=13 mutant cells). (c) Averaged amplitude of spontaneous [Ca2+]itransients of SAN myocytes in Tyrode’s solution (n=19 control,n=19 mutant cells), in ISO 2 nM (n=18,n=28 mutant cells) and ISO 100 nM (n=14 control,n=13 mutant cells). Perfusion with ISO reduced transient amplitude in mutant but not in control SAN cells (d). Statistics: two-way analysis of variance, followed by Sidak multiple comparisons test. (e) Histograms of caffeine-evoked (10 mM) Ca2+release (n=12 control,n=14 mutant cells,e-left) and decay (n=9 control,n=11 mutant cells,e-middle) in SAN myocytes.e-Right: Eeamples of line scan in control (top) and mutant (bottom) cell during caffeine application. Statistics: unpairedt-test; confocal images of spontaneously active control (f) and mutant (g) SAN myocytes loaded with Fluo-4 perfused with Tyrode’s solution (left) or 100 nM ISO (right). Red circle indicates [Ca2+]iwave; (h,i) averaged frequency of [Ca2+]iwaves (defined as a [Ca2+]irelease larger than 4 μm and/or with an intrinsic light intensity of >10% of the intensity measured during the following spontaneous [Ca2+]itransient) recorded in control and mutant SAN myocytes under Tyrode’s solution (n=12 control,n=11 mutant cells,h) and ISO 100 nM perfusion (n=12 control,n=11 mutant cellsi); (j,k) histograms comparing the averaged interval of the cycle length (CL) between two consecutive spontaneous [Ca2+]itransients preceding the wave and those between the wave and the following spontaneous [Ca2+]itransient (DAD) in Tyrode’s solution (n=11,j) and in ISO 100 nM (n=6,k) in mutant SAN myocytes. Statistics:t-test. *P<0.05, **P<0.01, ***P<0.001, ****P<0.0001. Error bars indicate s.e.m. Figure 5: [Ca 2+ ] i handling in I f –deficient SAN myocytes. ( a ) Averaged frequency of spontaneous [Ca 2+ ] i transients of SAN myocytes in Tyrode’s solution ( n =20 control, n =29 mutant cells), ISO 2 nM ( n =16 control, n =29 mutant cells) and in ISO 100 nM ( n =14 control, n =12 mutant cells). ( b ) Frequency of LCRs in Tyrode-perfused SAN myocytes ( n =19 control, n =24 mutant cells), in ISO 2 nM ( n =18 control and n =26 mutant cells) and ISO 100 nM ( n =14 control, n =13 mutant cells). ( c ) Averaged amplitude of spontaneous [Ca 2+ ] i transients of SAN myocytes in Tyrode’s solution ( n =19 control, n =19 mutant cells), in ISO 2 nM ( n =18, n =28 mutant cells) and ISO 100 nM ( n =14 control, n =13 mutant cells). Perfusion with ISO reduced transient amplitude in mutant but not in control SAN cells ( d ). Statistics: two-way analysis of variance, followed by Sidak multiple comparisons test. ( e ) Histograms of caffeine-evoked (10 mM) Ca 2+ release ( n =12 control, n =14 mutant cells, e -left) and decay ( n =9 control, n =11 mutant cells, e -middle) in SAN myocytes. e -Right: Eeamples of line scan in control (top) and mutant (bottom) cell during caffeine application. Statistics: unpaired t -test; confocal images of spontaneously active control ( f ) and mutant ( g ) SAN myocytes loaded with Fluo-4 perfused with Tyrode’s solution (left) or 100 nM ISO (right). Red circle indicates [Ca 2+ ] i wave; ( h , i ) averaged frequency of [Ca 2+ ] i waves (defined as a [Ca 2+ ] i release larger than 4 μm and/or with an intrinsic light intensity of >10% of the intensity measured during the following spontaneous [Ca 2+ ] i transient) recorded in control and mutant SAN myocytes under Tyrode’s solution ( n =12 control, n =11 mutant cells, h ) and ISO 100 nM perfusion ( n =12 control, n =11 mutant cells i ); ( j , k ) histograms comparing the averaged interval of the cycle length (CL) between two consecutive spontaneous [Ca 2+ ] i transients preceding the wave and those between the wave and the following spontaneous [Ca 2+ ] i transient (DAD) in Tyrode’s solution ( n =11, j ) and in ISO 100 nM ( n =6, k ) in mutant SAN myocytes. Statistics: t -test. * P <0.05, ** P <0.01, *** P <0.001, **** P <0.0001. Error bars indicate s.e.m. Full size image I f silencing induced bradycardia, AVBs and ventricular tachycardia in mutant mice To investigate the consequences of I f silencing in rhythmogenic centres in vivo , we performed telemetric electrocardiography (ECG) recordings in freely moving control and mutant mice. As western blot analysis of hHCN4-AYA protein indicated that the transgene expression reached a plateau after 5 weeks following DOX withdrawal (week 0), we continuously analysed the time course of ECG alterations for 8 weeks after induction of transgene expression following DOX withdrawal. HR of mutant mice constantly decreased and reached a plateau phase in week 6 ( Fig. 6a ). We did not record differences in the HR of control mice during the entire 6-week period (495±45 at week 0 and 508±49 beats min − 1 at week 6, n =3 P >0.05). At the same time, we observed a strong increase in the frequency of AVBs in mutant mice ( Fig. 6b ). The decrease in HR ( Fig. 6a ) and increase in the occurrence of conduction abnormalities ( Fig. 6b,c ) approximately paralleled the kinetics of hHCN4-AYA protein expression ( Fig. 1c ). To investigate the reversibility of the phenotype of mutant mice, we reintroduced DOX to the diet at the end of week 8 to repress transgene expression. After 4 weeks of DOX reintroduction, AVBs disappeared and the HRs of control and mutant mice were comparable ( Supplementary Fig. 9a,b ). Furthermore, voltage-clamp recordings of mutant SAN myocytes showed normalized cell capacitance and I f density 4–5 weeks after renewed administration of DOX to the food ( Supplementary Fig. 9c,d ). These observations demonstrate that the effects of hHCN4-AYA protein expression on HR are completely apparent after 5 weeks following DOX withdrawal and can be reversed by suppression of mutant subunit expression, indicating a causal relationship. 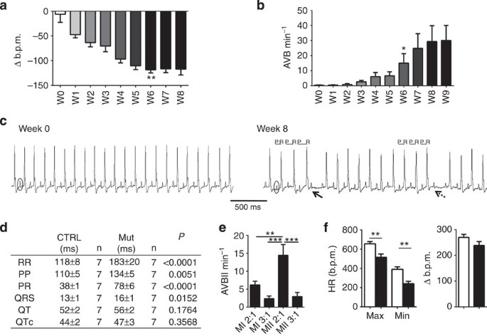Figure 6: Time course of HR slowing in mutant mice following DOX withdrawal. (a) Time course of the HR (in b.p.m.) slowing in mutant mice expressed as the difference in HR betweenn=3 control andn=5 mutant mice. DOX was removed from the diet at week 0 (W0). The maximum HR difference was observed at week 6 (from 525±16 b.p.m. at week 0 to 429±6 b.p.m. at week 6;ttest,P<0.001). (b) Relationship between the average increase in the number of AVB and the time elapsed after DOX withdrawal inn=5 mutant mice (0.2±0.2 AVB/60 s at week 0 versus 15±6 AVB/60 s at week 6;ttest,P<0.05). (c) Representative examples of ECG traces recorded from mutant mice before (left) and after (right) withdrawal of DOX. (d) Mean values of ECG intervals recorded from control and mutant mice. Statistics:t-test. (e) Averaged number of Mobitz type I and type II 2:1 (twoP-waves for one QRS complex) and 3:1 (threeP-waves for one QRS complex) AVBs during 30 s of ECG recording (n=9 mutant mice). (f-left) Averaged maximum and minimum HRs in control (open bars) and mutant (filled bars) mice. Statistics: two-way analysis of variance followed by Sidak multiple comparisons test. (f-right) Range of HR regulation calculated as differences between maximum and minimum HRs during continuous 24-h ECG recordings ofn=7 control andn=9 mutant mice (ttest,P>0.05). *P<0.05, **P<0.01, ***P<0.001. Error bars indicate s.e.m. Figure 6: Time course of HR slowing in mutant mice following DOX withdrawal. ( a ) Time course of the HR (in b.p.m.) slowing in mutant mice expressed as the difference in HR between n =3 control and n =5 mutant mice. DOX was removed from the diet at week 0 (W0). The maximum HR difference was observed at week 6 (from 525±16 b.p.m. at week 0 to 429±6 b.p.m. at week 6; t test, P <0.001). ( b ) Relationship between the average increase in the number of AVB and the time elapsed after DOX withdrawal in n =5 mutant mice (0.2±0.2 AVB/60 s at week 0 versus 15±6 AVB/60 s at week 6; t test, P <0.05). ( c ) Representative examples of ECG traces recorded from mutant mice before (left) and after (right) withdrawal of DOX. ( d ) Mean values of ECG intervals recorded from control and mutant mice. Statistics: t -test. ( e ) Averaged number of Mobitz type I and type II 2:1 (two P -waves for one QRS complex) and 3:1 (three P -waves for one QRS complex) AVBs during 30 s of ECG recording ( n =9 mutant mice). ( f -left) Averaged maximum and minimum HRs in control (open bars) and mutant (filled bars) mice. Statistics: two-way analysis of variance followed by Sidak multiple comparisons test. ( f -right) Range of HR regulation calculated as differences between maximum and minimum HRs during continuous 24-h ECG recordings of n =7 control and n =9 mutant mice ( t test, P >0.05). * P <0.05, ** P <0.01, *** P <0.001. Error bars indicate s.e.m. Full size image ECG recordings of mutant mice deprived of DOX after weaning showed that I f silencing induced multiple and severe alterations in HR and rhythm. SAN activity of mutant mice was characterized by a prolonged SAN rate (PP intervals) and the presence of SAN pauses. Ventricular (RR) beating rates of mutant mice were also considerably lower in comparison with control animals ( Fig. 6d ). We recorded strongly prolonged atrioventricular conduction (PR) intervals in mutant mice ( Fig. 6d ). Both Mobitz type I and II AVBs were observed in mutant mice, but the frequency of type II Mobitz AVBs was higher than that of type I AVBs ( Fig. 6e ). During a 24-h recording period, maximum and minimum HRs were lower in mutant than in control mice, but the absolute difference between maximum and minimum HRs did not differ, showing a preserved degree of HR regulation ( Fig. 6f ). Consistent with the prominent effect of hHCN4-AYA expression on PF myocyte rhythmicity and DAD occurrence ( Fig. 4 ), mutant mice also showed prolonged QRS complexes and frequent episodes of ventricular tachycardia in comparison with control mice (see below). Ventricular repolarization (QT and QTc intervals) was not affected in mutant mice ( Fig. 6d ). As chronic bradycardia often goes along with cardiac hypertrophy [35] , we investigated whether long-term transgene expression and bradycardia led to changes in left ventricular size and function in mutant mice. In line with telemetric recordings, ecocardiography showed slower HRs in mutant mice, but normal left ventricular and atrial mass to body weight ratios ( Supplementary Fig. 10 ). Left ventricular end-diastolic volume, stroke volume and area shortening under control and stimulated conditions did not differ between control and mutant mice ( Supplementary Fig. 10 ). Recordings showed a tendency towards a reduced cardiac output in mutant mice, but this difference did not reach statistical significance ( Supplementary Fig. 10 ). Furthermore, mutant mice did not show alterations in blood pressure measured by means of radiotelemetry as a function of locomotor activity in the home cage ( Supplementary Fig. 11 ). HR of mutant mice was insensitive to the I f inhibitor ivabradine To investigate whether I f silencing in mutant mice corresponded to the elimination of the pharmacological sensitivity of HR to I f inhibition, we recorded ECGs of control and mutant mice on injection of ivabradine (IVA), a selective I f inhibitor [36] . Administration of IVA (6 mg kg −1 ) reduced the HR in control, but not in mutant mice ( Fig. 7a,b ). No IVA effect was detected in mutant mice when considering the ventricular (RR interval, Fig. 7b ) or SAN rates (PP interval, Fig. 7c ). Remarkably, HRs and SAN rates of IVA-treated control mice and untreated mutant mice were similar ( Fig. 7d ), indicating that the negative chronotropic effect of IVA was completely abolished. Likewise, IVA had no effect in isolated spontaneously beating right atrial preparations from mutant mice ( Supplementary Fig. 12 ), but it caused a slowly developing, concentration-dependent decrease in spontaneous beating rates in control atria, which were comparable to those observed in mutant SAN myocytes perfused with ISO ( Supplementary Figs 12 and 13 ). In agreement with these results, IVA slowed pacemaker activity of isolated control SAN myocytes by ~33% but did not affect the spontaneous beating rate of mutant myocytes ( Fig. 7e ). These observations indicate that no residual, physiologically relevant I f current was present in hCN4-AYA-expressing mutant SAN myocytes. 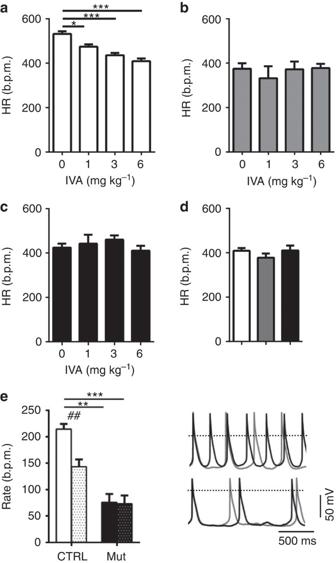Figure 7: Loss of ivabradine-mediated HR reduction in mutant mice. Dose–response relationship of HR (RR) to intraperitoneal administration of IVA inn=13 control (a) andn=7 mutant (b) mice (analysis of variance (ANOVA) followed by Tukey’s multiple comparisons test). (c) Averaged SAN rate (PP interval) in mutant mice after IVA administration. (d) Comparison between the SAN rate of control (white bar) and mutant (black bar) mice as compared with the ventricular rate of mutant mice (grey bar) after injection of the highest dose of IVA (6 mg kg−1, ANOVA followed by Tukey’s multiple comparisons test). (e-left) Averaged spontaneous beating rates of SAN myocytes, isolated fromn=9 control (white bars) andn=8 mutant mice (black bars), in Tyrode’s solution (empty bars) and after perfusion with ivabradine (1 μM, dotted bars). Statistics: two-way ANOVA followed by Sidak multiple comparisons test.##P<0.01, *P<0.05, **P<0.01, ***P<0.001. Error bars define the s.e.m. (e-right) Sample action potentials recorded from control (top) and mutant (bottom) SAN myocytes before (black line) and after (grey line) application of 1 μM IVA. Figure 7: Loss of ivabradine-mediated HR reduction in mutant mice. Dose–response relationship of HR (RR) to intraperitoneal administration of IVA in n =13 control ( a ) and n =7 mutant ( b ) mice (analysis of variance (ANOVA) followed by Tukey’s multiple comparisons test). ( c ) Averaged SAN rate (PP interval) in mutant mice after IVA administration. ( d ) Comparison between the SAN rate of control (white bar) and mutant (black bar) mice as compared with the ventricular rate of mutant mice (grey bar) after injection of the highest dose of IVA (6 mg kg −1 , ANOVA followed by Tukey’s multiple comparisons test). ( e -left) Averaged spontaneous beating rates of SAN myocytes, isolated from n =9 control (white bars) and n =8 mutant mice (black bars), in Tyrode’s solution (empty bars) and after perfusion with ivabradine (1 μM, dotted bars). Statistics: two-way ANOVA followed by Sidak multiple comparisons test. ## P <0.01, * P <0.05, ** P <0.01, *** P <0.001. Error bars define the s.e.m. ( e -right) Sample action potentials recorded from control (top) and mutant (bottom) SAN myocytes before (black line) and after (grey line) application of 1 μM IVA. Full size image Autonomic nervous system activity modulated the functional impact of I f silencing on HR and impulse conduction We then investigated the impact of I f silencing on in vivo HR regulation. Pharmacological inhibition of the sympathetic branch of the autonomic nervous system by propranolol (5 mg kg −1 ) significantly decreased the HRs of control mice, but had no effect on those of mutant mice ( Fig. 8a ). Propranolol reduced the HR of control mice to levels that did not differ from those of mutant mice, either under basal conditions or in the presence of propranolol ( Fig. 8a ). Likewise, combined injection of propranolol and atropine (0.5 mg kg −1 ), an inhibitor of the parasympathetic input, did not significantly affect the HR of mutant mice ( Fig. 8b ). Interestingly, pharmacological inhibition of the autonomic input by combined injection of atropine and propranolol strongly reduced the number of AVBs in mutant mice ( Fig. 8c,d ). These observations indicate that the physiological impact of I f silencing on HR determination and impulse conduction was reduced in the absence of autonomic input. 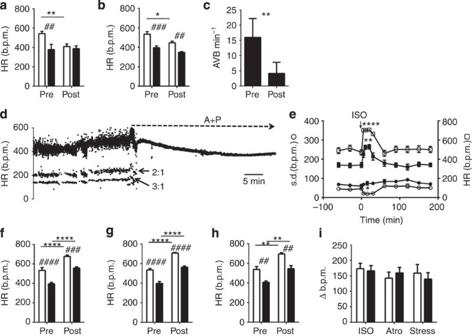Figure 8: Autonomic regulation of HR and impulse conduction in mutant mice. Averaged HR recorded fromn=11 control (open bars) andn=11 mutant (filled bars) mice before (pre) and after (post) intraperitoneal injection of propranolol (a), or atropine and propranolol (b). Statistics inaandb: two-way analysis of variance (ANOVA) followed by Sidak multiple comparisons test. (c) Number of AVBs measured in a 30-s window every 5 min for a 30-min total recording period before (pre) and after (post) injection. AVB counting started 30 min after injection to allow the effect to stabilize. Statistics:t-test. (d) Sample dot plot of beat-to-beat variability (b.p.m.) of HR of mutant mice before and after (dotted line) injection of atropine and propranolol. Note the slow ventricular beats in the presence of AVB before injection. Arrows indicate AVBs (twoP-waves for one QRS complex, 2:1; threeP-waves for one QRS complex, 3:1). (e) Time course of HR and the s.d. of HR before and after injection of ISO. (f–h) HR in control and mutant mice before and after injection of atropine (f) or ISO (g) inn=8 control andn=12 mutant mice. (h) HR before and after 5-min swimming test, inn=5 control (open bars) andn=7 mutant (filled bars) mice. (i) Delta of HR following different β-adrenergic stimulations. Values represent the mean difference between pre- and post-adrenergic pathway activation (pharmacological or physiological). Statistics: two-way ANOVA followed by Sidak multiple comparisons test. *P<0.05, **P<0.01, ***P<0.001, ****P<0.0001,##P<0.01,###P<0.001,####P<0.0001. Error bars indicate s.e.m. Figure 8: Autonomic regulation of HR and impulse conduction in mutant mice. Averaged HR recorded from n =11 control (open bars) and n =11 mutant (filled bars) mice before (pre) and after (post) intraperitoneal injection of propranolol ( a ), or atropine and propranolol ( b ). Statistics in a and b : two-way analysis of variance (ANOVA) followed by Sidak multiple comparisons test. ( c ) Number of AVBs measured in a 30-s window every 5 min for a 30-min total recording period before (pre) and after (post) injection. AVB counting started 30 min after injection to allow the effect to stabilize. Statistics: t -test. ( d ) Sample dot plot of beat-to-beat variability (b.p.m.) of HR of mutant mice before and after (dotted line) injection of atropine and propranolol. Note the slow ventricular beats in the presence of AVB before injection. Arrows indicate AVBs (two P -waves for one QRS complex, 2:1; three P -waves for one QRS complex, 3:1). ( e ) Time course of HR and the s.d. of HR before and after injection of ISO. ( f – h ) HR in control and mutant mice before and after injection of atropine ( f ) or ISO ( g ) in n =8 control and n =12 mutant mice. ( h ) HR before and after 5-min swimming test, in n =5 control (open bars) and n =7 mutant (filled bars) mice. ( i ) Delta of HR following different β-adrenergic stimulations. Values represent the mean difference between pre- and post-adrenergic pathway activation (pharmacological or physiological). Statistics: two-way ANOVA followed by Sidak multiple comparisons test. * P <0.05, ** P <0.01, *** P <0.001, **** P <0.0001, ## P <0.01, ### P <0.001, #### P <0.0001. Error bars indicate s.e.m. Full size image I f silencing did not impair maximal β-adrenergic regulation of HR We then assessed the capability of mutant mice to increase their HR under conditions of maximal sympathetic input, that is, direct pharmacological stimulation of β-adrenergic receptors or physical exercise. Injection of ISO or atropine similarly increased the HR in both control and mutant mice ( Fig. 8e–g ). Contrary to the inhibition of the autonomic nervous system ( Fig. 8d ), ISO did not reduce cardiac dysrhythmia due to SAN pauses and AVBs ( Fig. 8e ). Comparable results were obtained from ISO-stimulated, spontaneously beating right atria preparations ( Supplementary Fig. 10c ). Although the maximum HR in ISO-stimulated mutant mice did not reach that of control mice ( Fig. 8f ), the relative extent of ISO-induced increase did not differ between the two strains ( Fig. 8h ). Likewise, during a swimming test combining mental stress with physical activity ( Fig. 8g,h ), the HR was increased to an extent similar to that in control mice. Taken together, these data show that in spite of complete I f silencing the autonomic nervous system was still capable of regulating HR ( Fig. 8i ). Genetic inactivation of GIRK4 channels ameliorated SAN failure, atrioventricular dysfunction and ventricular arrhythmia in mutant mice As the impact of I f silencing on HR and atrioventricular dysfunction depended on the status of the autonomic nervous system, we investigated the possibility of counterbalancing I f loss-of-function in mutant mice by reducing the influence of the parasympathetic nervous system on HR and atrioventricular conduction. We thus crossed mutant mice with GIRK4 ( Kir3.4 ) knockout mice ( GIRK4 −/− ) deficient in the cardiac G-protein-gated inwardly rectifying K + current I KACh [37] to obtain double-mutant Mut/ GIRK4 −/− mice. Telemetric 24-h ECG recordings in Mut/ GIRK4 −/− mice showed a higher HR in comparison with mutant animals, although the mean RR interval measured in double-mutant mice was still significantly longer than that of controls ( Fig. 9a ). The SAN rates (PP interval) of Mut/ GIRK4 −/− and of mutant mice did not differ from each other ( Fig. 9b ). However, SAN pauses were absent in Mut/ GIRK4 −/− mice, indicating that GIRK4 loss-of-function improved SAN function. The PR interval was significantly shorter in Mut/ GIRK4 −/− mice, although it was still longer than that in control mice ( Fig. 9c ). The occurrence of AVBs was drastically reduced in Mut/ GIRK4 −/− , suggesting that the activity of GIRK4 channels in the AVN contributed to conduction dysfunction in mutant mice ( Fig. 9d ). Loss of GIRK4 channels did not normalize QRS intervals, which were similarly prolonged in Mut/ GIRK4 −/− and mutant mice ( Fig. 9e ). In most cases, the ventricular tachycardia/tachyarrhythmia observed in mutant mice was preceded by dysfunction of atrial rhythm or AVBs. In particular, SAN pauses and AVBs preceded ventricular tachycardia in >70% of cases, suggesting a causal relationship ( Fig. 9j ). In line with the absence of SAN pauses and AVBs in Mut/ GIRK4 −/− mice, we did not record ventricular tachycardia or extrasystoles in these animals ( Fig. 9k , Table 1 ). Similar to control and mutant mice, Mut/ GIRK4 −/− animals showed a preserved degree of HR regulation and a normal recovery of resting HR following direct β-adrenergic stimulation ( Supplementary Fig. 13 ). These data indicate that the inactivation of GIRK4 channels was effective in improving SAN automaticity and atrioventricular conduction, and in preventing ventricular arrhythmias in I f -deficient mice ( Table 1 ). 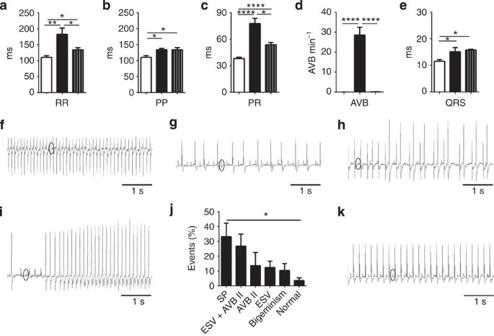Figure 9: Improvement of HR in mutant mice byGIRK4gene knockout. Averaged RR (a), PP (b), PR (c), number of AVBs (d) and QRS (e) inn=7 control (white bar),n=7 mutant (black bar) andn=8 Mut/GIRK4−/−(black bar with white stripes) mice. Statistics (a–e): analysis of variance (ANOVA) followed by Tukey’s multiple comparisons test. *P<0.05, **P<0.01, ****P<0.0001. Error bars define the s.e.m. (f) Representative example of ECG recordings from control mice. (g–i). Different examples of ECG recordings showing HR dysfunction recorded from mutant mice. (g) Second-degree AVB; (h) ventricular extrasystoles; (i) ventricular tachycardia. (j) Relative percentages of SAN or AVN dysfunctions preceding a period of ventricular tachycardia inn=5 mutant mice (SP, sinus pauses; ESV, ventricular extrasystoles). (k) ECG recorded from Mut/GIRK4−/−mice. Small circles indicateP-waves. Figure 9: Improvement of HR in mutant mice by GIRK4 gene knockout. Averaged RR ( a ), PP ( b ), PR ( c ), number of AVBs ( d ) and QRS ( e ) in n =7 control (white bar), n =7 mutant (black bar) and n =8 Mut/ GIRK4 −/− (black bar with white stripes) mice. Statistics ( a – e) : analysis of variance (ANOVA) followed by Tukey’s multiple comparisons test. * P <0.05, ** P <0.01, **** P <0.0001. Error bars define the s.e.m. ( f ) Representative example of ECG recordings from control mice. ( g – i ). Different examples of ECG recordings showing HR dysfunction recorded from mutant mice. ( g ) Second-degree AVB; ( h ) ventricular extrasystoles; ( i ) ventricular tachycardia. ( j ) Relative percentages of SAN or AVN dysfunctions preceding a period of ventricular tachycardia in n =5 mutant mice (SP, sinus pauses; ESV, ventricular extrasystoles). ( k ) ECG recorded from Mut/ GIRK4 −/− mice. Small circles indicate P -waves. Full size image Table 1 Summary table of the fraction of CTRL, Mut or Mut/ GIRK4 −/− mice with heart rhythm disturbances. Full size table Cardiac pacemaker activity is a complex phenomenon requiring the interaction of different classes of membrane ion channels [1] , [Ca 2+ ] I cycling [38] and probably other mechanisms yet to be identified. The ‘funny’ current I f is thought to play a key role in the generation and regulation of automaticity in the adult heart [8] , but its functional role and importance are still incompletely understood [9] , [21] . Pharmacological [39] and genetic studies in humans [16] , [17] , [18] , [19] indicate a role for I f in the determination of HR and rhythm. However, a body of data obtained from mouse models in which HCN4 subunits were deleted showed contrasting results in relation to the importance of these channels in SAN pacemaking and impulse conduction [21] , [22] , [23] . Furthermore, although several groups described the phenotype of mice deficient in HCN1 (ref. 15 ), HCN2 (ref. 40 ) or HCN4 (refs 21 , 23 , 41 ) subunits, no mouse model has yet been available that shows a suppression of I f conductance of up to >95% of its control value. In this study, we show for the first time heart-specific and time-controlled silencing of I f conductance in both the SAN and the conduction system. We show that chronic functional ablation of I f conductance induces severe abnormalities of both atrial and ventricular rhythms by altering Ca 2+ handling in pacemaker myocytes. The resulting complex cardiac arrhythmia was prevented by inactivation of GIRK4 channels. We used the Tet-off strategy to express mutant hHCN4-AYA non-conducting subunits to suppress f -channel conductance in a dominant-negative manner. Using this experimental approach, we achieved I f silencing without deletion of HCN-channel subunits from the plasma membrane and thus without depletion of HCN-associated proteins. Embryonic lethality observed when mutant hHCN4-AYA channels are expressed during embryonic development suggests that I f conductance is required for the embryonic heart to be viable ( Fig.1 ), which is compatible with the phenotype of both global and heart-specific HCN4 knockout mice [26] . Western blotting experiments demonstrated that the hHCN4-AYA protein was highly expressed in the atria and ventricles of adult mutant mice ( Fig.1 ). Similar to findings from immunostainings of native HCN4 channels of SAN and AVN preparations ( Fig. 2 ), or of isolated myocytes, for hHCN4-AYA protein ( Supplementary Fig. 5 ) indicated that the mutant channel protein was targeted to the cell membrane. Consistent with the immunostaining in mutant pacemaker tissue and the dominant-negative effect on HCN4- and HCN2-mediated currents by hHCN4-AYA recorded in Xenopus oocytes, I f was abolished at voltages spanning the diastolic depolarization range of myocytes from the SAN and the conduction system ( Fig. 3 ). I f silencing throughout the conduction system suggested that mutant hHCN4-AYA channels exerted a dominant-negative effect, also on native HCN1 channels. In agreement with the complete silencing of I f , pacemaker activity of mutant SAN myocytes, intact atrial preparations and the in vivo HR of hHCN4-AYA mutant mice were insensitive to IVA ( Fig. 7 and Supplementary Fig. 12 ). The reasons for the increase in cell membrane capacitance in mutant myocytes are unclear at present. As mutant and Mut/ GIRK4 −/− SAN myocytes showed similar membrane capacitance ( Supplementary Fig. 6 ), we can exclude that this phenomenon is due to cellular hypertrophy secondary to chronic AVBs. We thus speculate that the increase in cell size in mutant myocytes represents an adaptive mechanism to increased SR Ca 2+ load ( Fig. 5 ). Action potential recordings of myocytes from the heart-rhythmogenic centres and Ca 2+ imaging of mutant SAN myocytes showed that I f silencing had strong effects on pacemaker activity and [Ca 2+ ] i handling in these cells. Mutant myocytes displayed slow diastolic depolarization ( Fig. 4a,e,i ) and a high incidence of DADs ( Fig. 4c,g,k ). hHCN4-AYA expression induced a 76% reduction in the basal spontaneous beating rate in SAN myocytes, 51% in AVN and 67% in PF myocytes ( Fig. 4 ). β-Adrenergic activation by ISO abolished the differences in action potential amplitude and duration between control and mutant SAN and AVN myocytes ( Supplementary Table 1 ). We attribute these differences to a partial loss of Ca 2+ -activated SK channel activity [42] secondary to low cellular spontaneous beating rate, which induces low rate-dependent opening of Ca v 1.3 channels [43] . Perfusion of ISO stimulates Ca v 1.3 channels [44] and could also activate mERG1 channels, thereby normalizing action potential duration [45] . The increased SR Ca 2+ load in mutant SAN myocytes induced spontaneous, partially synchronized openings of RYRs, thereby forming [Ca 2+ ] i waves [34] ( Fig. 5 ). It is well established that SR Ca 2+ overload-mediated [Ca 2+ ] i waves activate the Na + /Ca 2+ exchanger, thus depolarizing the membrane potential and causing DADs [46] . Consistent with this view, DADs in mutant SAN myocytes were generated by spontaneous [Ca 2+ ] i waves, presumably because of SR Ca 2+ overload ( Fig. 5e ). Such a mechanism would also explain the increased frequency of spontaneous [Ca 2+ ] i sparks recorded in mutant myocytes ( Fig. 5e ). Two non-mutually exclusive phenomena may account for SR Ca 2+ overload in mutant SAN myocytes. First, mutant myocytes showed augmented density of peak I Ca,L ( Supplementary Fig. 7 ) translating into increased Ca 2+ entry during the action potential upstroke and Ca 2+ uptake in the SR during the decaying phase of the [Ca 2+ ] i transient. Second, the slow diastolic phase of mutant myocytes can increase the SR Ca 2+ load via longer sarcoplasmic reticulum Ca 2+ ATPase -mediated Ca 2+ uptake before an action potential eventually occurs. Although β-adrenergic activation by ISO increased pacemaker activity, the difference in spontaneous beating rate between control and mutant myocytes was still 61% in SAN, 43% in AVN and 42% in PFs ( Fig. 4 ). These observations are consistent with data on Ca 2+ handling. Even though ISO appeared to facilitate ryanodine receptor-dependent Ca 2+ release, it only incompletely normalized spark frequency and SR Ca 2+ overload. Similarly, ISO did not reduce DADs or [Ca 2+ ] i waves in mutant myocytes ( Figs 4 and 5 ). Although we did not directly investigate the mechanistic link between [Ca 2+ ] i waves and delayed formation of the following pacemaker action potential under ISO, previous work by us and another group indicates that diminished SR Ca 2+ load delays the formation of spontaneous [Ca 2+ ] i transients [47] and that Ca 2+ uptake is directly linked to the rate of pacemaking in rabbit SAN myocytes [48] . It is possible that [Ca 2+ ] i waves drive the SR into a partially depleted state, thus preventing rapid generation of the following pacemaker impulse. Taken together, our data demonstrate that I f silencing impairs pacemaker activity of automatic myocytes by eliminating f -channel activity in the diastolic depolarization, which leads to altered [Ca 2+ ] i release and Ca 2+ handling. Consistent with I f silencing in the three main rhythmogenic centres of the heart, in vivo HR of mutant mice was reduced by 36%. Mutant mice displayed a significant reduction in SAN activity, which was reflected in frequent pauses and an 18% slowing of the SAN rate ( Fig. 6 and Table 1 ), a value that matches that recorded in healthy human volunteers treated with the I f blocker IVA [39] . In spite of significant SAN dysfunction, we did not find evidence of a reduction in the sympathetic regulation of HR in hHCN4-AYA mutant mice. Indeed, spontaneously beating myocytes ( Fig. 4 ), intact atrial preparations ( Supplementary Fig. 12 ) or in vivo HR ( Fig. 6 ) showed a preserved degree of regulation. Likewise, the relative increase in HR after injection of atropine, ISO, or following stress did not differ between control and mutant mice, demonstrating that the compliance of the sympathetic regulation of HR was preserved under conditions of I f silencing ( Fig. 7 ). We attribute the preserved HR regulation in mutant mice to the capability of β-adrenergic activation to partially increase ryanodine receptor-dependent Ca 2+ release [49] , [50] in mutant SAN myocytes ( Fig. 5 ), as well as to stimulation of other mechanisms involved in automaticity such as I Ca,L [44] and Ca 2+ /calmodulin-dependent kinase II [51] . Although I f silencing obviously did not impair maximum β-adrenergic regulation of pacemaking, our data show that the importance of I f in the determination of in vivo HR and atrioventricular conduction was dependent on the activity of the autonomic nervous system. Indeed, pharmacological inhibition of the β-adrenergic tone by propranolol abolished the difference in basal HR between control and mutant mice ( Fig. 8 ). Likewise, the ‘intrinsic’ in vivo HR measured on combined administration of atropine and propranolol did not significantly differ between control and mutant mice ( Fig. 8b ), which is consistent with our previous finding that inhibition of the autonomic nervous system input did not affect the HR of mice with conditional abolition of cAMP-dependent I f regulation [52] . These observations suggest that in freely moving mice the establishment of resting HR in vivo by the autonomic nervous system involves I f . In comparison, the setting of intrinsic HR under conditions of autonomic nervous system inhibition is less dependent on f -channel activity. The finding of similar intrinsic SAN rates measured ex vivo in isolated control and in mutant atrial preparations is in line with this concept ( Supplementary Fig. 12 ). However, isolated atrial preparations are mechanically unloaded, while blood flow-induced mechanical forces cyclically challenge the SAN in vivo . Thus, it is possible that mechano-electric feedback in SAN myocytes or fibroblasts [53] contributes to pacemaking in vivo , especially under conditions of I f silencing. The similar spontaneous beating rate of control and mutant atria is likely to be due to the combined compensatory effects of the well-known phenomenon of ‘pacemaker shift’ of the dominant pacemaker site within the SAN [54] to a region that is less sensitive to I f silencing [55] , and to the augmented I Ca,L density in mutant SAN myocytes ( Supplementary Fig. 7 ). A shift of the leading pacemaker site in vivo may also explain, at least in part, the different effects of hHCN4-AYA expression on the pacemaker activity in SAN myocytes in vitro and on the SAN in vivo (PP interval). Joung et al . [56] have reported that DADs that fail to trigger a local action potential prevent the subsequent SAN activation in intact SAN preparations. We thus propose that [Ca 2+ ] i wave-induced DADs recorded in mutant SAN myocytes underlie SAN pauses recorded in vivo . Furthermore, the delay in the coupling time between a DAD and the following action potential is an additional mechanism explaining SAN pauses and bradycardia in mutant mice. SAN bradycardia in mutant mice was always accompanied by strongly impaired atrioventricular conduction. The PR interval of conducted SAN impulses was almost double of that in control animals, and all mice investigated showed a high frequency in second-degree AVBs ( Fig. 8 ). Some mutant mice exhibited a complete uncoupling of atrial and ventricular rhythms (third-degree block), which demonstrates that I f activity is also critical for impulse conduction through the AVN. Consistent with the prominent effect of hHCN4-AYA expression in pacemaking of PF myocytes, mutant mice showed a significantly (19%) prolonged QRS complex. Some mutant mice exhibited ventricular extrasystoles and episodes of ventricular tachycardia ( Fig. 9 ). Similar to SAN, both mutant AVN and PF myocytes showed a high incidence of DADs. These DADs may underlie AVBs by preventing AVN activation and inducing ventricular extrasystoles and tachycardia. In this context, modelling studies suggest that a limited number of myocytes developing synchronous DADs is sufficient to trigger premature ventricular contraction and arrhythmia in PF [57] . Our observation of ventricular arrhythmia in mutant mice is compatible with a previous case report showing ventricular tachycardia in a patient with a genetic loss-of-function of HCN4 (ref. 20 ). As HCN3 channels have been proposed to regulate ventricular repolarization [58] , mutant hHCN4-AYA channels may also induce arrhythmogenic DADs in ventricular myocytes by exerting a dominant-negative effect on native HCN3 subunits. In contrast to what was reported in cardiac-specific HCN4 knockout mice (ci-HCN4-KO) [23] , we did not observe lethal heart block in mutant mice. In mutant mice with complete AV block, a viable ventricular idiopathic rhythm persisted, suggesting that the His-Purkinje network was still able to generate sufficient automaticity in spite of I f silencing. Both Baruscotti et al . [23] and our group used αMHC promoter lines. It is thus unlikely that the difference between ciHCN4-KO and HCN4-AYA mutant mice is due to differential efficiency of Cre -mediated inactivation of HCN4 alleles [23] versus expression of hHCN4-AYA transgene in the conduction system described here. It is possible, although, that idioventricular rhythm deficiency in ci-HCN4-KO mice is a consequence of a fast Cre -mediated loss of HCN4 protein versus more slowly progressing hHCN4-AYA-mediated I f silencing in mutant mice. Another hypothesis is that idioventricular rhythm requires intact HCN4 protein. We did not observe atrioventricular dysfunction in control mice treated with IVA. We hypothesize that IVA does not impair impulse conduction because of its use-dependent properties of block, which predicts that the drug dissociates from f -channels at low SAN beating rates [59] . Genetic inactivation of I KACh by GIRK4 gene knockout effectively prevented SAN pauses, AVBs and ventricular tachycardia in mutant mice ( Fig. 9 ). I KACh slows diastolic depolarization [60] and atrioventricular conduction [61] in the mouse heart. As the membrane voltage of mutant pacemaking myocytes is characterized by slow diastolic depolarization and a high incidence of DADs, it is tempting to speculate that I KACh activation favours DAD formation in mutant mice in vivo . In contrast, in the absence of I KACh , a significant fraction of DADs would elicit a normal action potential in Mut/ GIRK4 −/− mice, thus abolishing SAN pauses and facilitating AVN activation and conduction. The improved SAN activity and impulse conduction in turn may suppress arrhythmogenic DADs in PFs of Mut/ GIRK4 −/− mice. The presence of such a mechanism is supported by the observation that the vast majority of episodes of ventricular tachycardia are preceded by SAN pauses or AVBs ( Fig. 9 ). In addition, PF myocytes may develop fully conducted action potentials rather than arrhythmogenic DADs in the absence of I KACh in vivo . Our results demonstrate that I f is an important mechanism effective in counterbalancing the negative dromotropic effect of I KACh activation in AVN, and show that f -channels provide AVN myocytes with a critical inward current under physiological conditions. It is an interesting observation that both mutant and Mut/ GIRK4 −/− mice show a preserved degree of HR regulation, as well as normal recovery of resting HR ( Supplementary Fig. 13 ). This last observation suggests that the delayed recovery of the resting HR, which is typically present in GIRK4 −/− (ref. 60 ) mice, is linked to I f activity. It is an attractive hypothesis that pharmacological inhibition of GIRK4 channels in the heart may be used to restore atrioventricular dysfunction in patients with AVB due to loss-of-function of ion channels involved in cardiac conduction. Cloning of HCN constructs Murine HCN4 and HCN2 (mHCN4 and mHCN2) and human HCN4 (hHCN4) complementary DNAs (GenBank Acc. NM_001081192, NM_008226 and NM_005477) in pCDNA1 vector were kindly provided by Benjamin Kaupp (Forschungszentrum caesar, Bonn, Germany). A HA epitope tag (YPYDVPDYA) was attached to the N terminus of the open-reading frame of hHCN4 (ref. 19 ). The selectivity filter GYG motif was mutated to AYA by overlap PCR-based, site-directed mutagenesis resulting in hHCN4-G480A/G482A (hHCN4-AYA). For two-electrode voltage-clamp experiments, mHCN4, mHCN2 and HA-hHCN4-AYA were cloned into an RNA expression vector (pGem-HeJuel [62] ). For the generation of transgenic mice, the Tet-responsive element (Tre-Tight) of pTRE-Tight (Clontech, Mountain View, CA, USA) was cloned into pWHERE2 v.01 (Invivogen, San Diego, CA, USA). HA-hHCN4-AYA was inserted downstream of Tre. All coding sequences were verified by direct sequencing. Two-electrode voltage-clamp experiments in Xenopus oocytes Xenopus oocytes were obtained from tricaine-anaesthetized animals. Ovaries were treated with collagenase (3 mg ml −1 , Sigma-Aldrich Chemie GmbH, Taufkirchen, Germany) in OR2 solution (in mM: NaCl 82.5, KCl 2, MgCl 2 1, HEPES 5, pH 7.4) for 2–3 h and subsequently stored in gentamycin solution (in mM: NaCl 75, KCl 2, CaCl 2 2, MgCl 2 1, HEPES 5, pH 7.4) with additional Na pyruvate (550 mg l −1 ) and gentamycin (50 mg l −1 ) at 18 °C. Oocytes were injected with cRNA (in ng)-encoding mHCN4 (1.0 or 0.5), mHCN2 (0.2 or 0.1) and HA-hHCN4-AYA (1.0 or 0.2). The effect of HA-hHCN4-AYA on mHCN4 and mHCN2 was tested by coexpression of the two constructs with the pore mutant at a 1:1 ratio. Standard two-electrode voltage-clamp recordings were performed at room temperature (RT; 21–23 °C) 3 days after injection. ND66 solution (in mM: NaCl 66, KCl 32, CaCl 2 1.8, MgCl 2 1, HEPES 5, pH 7.4) was used as a perfusion solution [63] . The pipette solution contained 3 M KCl. Generation of mutant transgenic mice Transgenic mice carrying the pWHERE-Tre-HA-hHCN4-AYA (C57BL/6J-Tg(tetO-hHCN4-AYA) CIsb) construct were generated by pronuclear injection using standard techniques. Founder mice and the resulting offspring were genotyped by PCR (primers: 5′- GGCATGTCCGACGTCTGGCTCAC -3′ and 5′- TCACGAAGTTGGGGTCCGCATTGG -3′) using ear or tail biopsies and crossed with heart-specific promoter transgenic mice (C57BL/6J -Tg(Myh6-tTA)6Smbf/J) [25] , which were obtained from the Jackson Laboratories (Bar Harbor, MA, USA) and backcrossed to the C57BL/6J background for more than seven generations. These mice are referred to as mutant (Mut) mice. To investigate the consequences of I f silencing in PF cells, mutant mice (C57BL/6J-Tg(Myh6-tTA, tetO-hHCN4-AYA) were crossed with heterozygous knockin mice in which EGFP was knocked in the gene coding for Cx40 ( Cx40 +/tm(EGFP)Lumi ) [31] to give rise to triple-transgenic C57BL/6J-Tg(Myh6-tTA, tetO-hHCN4-AYA, Cx40 +/tm(EGFP) (short: Mut/ Cx40 +/EGFP ) mice. To generate double-transgenic mutant mice that are also GIRK4 deficient (Mut/ GIRK4 −/− ) , double-transgenic mutant mice were crossbred with GIRK4 −/− mice [37] . Care and use of animals Mixed genotype groups of each gender of no more than five animals were housed in standard mouse cages under specific pathogen-free conditions (12:12-h dark–light cycle, constant temperature, constant humidity and food and water ad libitum ). Double-transgenic mutant mice and their tTA transgenic control littermates received either normal food or food drugged with 50 mg kg −1 DOX hydrochloride (Ssniff Spezialdiäten, Soest, Germany; Graymor Chemical, Hamburg, Germany) when breeding pairs were set up. Care and use of animals and experimental procedures were in accordance with the German Law for the Protection of Animals and approved by the Ministry of Science and Public Health of the City State of Hamburg, Germany. The study conforms to the Guide for the Care and Use of Laboratory Animals published by the US National Institutes of Health (NIH Publication No. 85–23, revised 1996) and to European directives (86/609/CEE). Protein isolation and western blotting Frozen hearts from 10-week-old male mice were pulverized in liquid nitrogen and homogenized in 10% glycerol, 3% SDS and 62.5 mM Tris (pH 6.8) containing a protease inhibitor mix (Sigma-Aldrich Chemie GmbH, Taufkirchen, Germany). Proteins were fractionated on NuPAGE 4–12% Bis-Tris gels (Invitrogen) in NuPAGE MOPS SDS running buffer (Invitrogen) and electrophoretically transferred to PROTRAN nitrocellulose membranes (Whatman GmbH, Dassel, Germany). Western blotting analysis was performed according to standard methods. Antibodies against the HA epitope tag (3F10 (Roche, Basel, Switzerland), 1:500 dilution) and calsequestrin (Affinity BioReagents, Golden, CO, USA) 1:2,500 dilution) were used as primary antibodies. Staining of intact SAN–AVN preparations and isolated myocytes Whole-mount immunofluorescence: Mouse heart nodal tissue was dissected from the right atrium, including the SAN and AVN regions, and fixed at 4 °C for 20 min with 4% paraformaldehyde. Fixed tissue was washed for 30 min in PBS at 4 °C and incubated for 30 min with 10% goat serum and 1% mouse blocking reagent (Vectashield) in PBS/0.1% Triton X-100. Subsequent incubation with primary antibodies was carried out overnight at 4 °C in mouse monoclonal anti-HA (1/100, clone 12C5A, DSHB Univ. Iowa) and rabbit polyclonal anti-HCN4 (1/200, Alomone), or rabbit polyclonal anti-HCN1 (1/200, Alomone) diluted in PBS/0.1% TritonX100. After rinsing in PBS-TX100, tissue was further incubated at 37 °C for 1 h using a 1/100 dilution of secondary Alexa488-conjugated anti-mouse IgGs and Alexa555-conjugated anti-rabbit IgGs, both from Molecular Probes (InVitrogen, Saint Aubin, France). After rinsing with PBS/Triton X-100, tissue was briefly treated with Sudan Black (Sigma, 3% in 70% ethanol) to quench autofluorescence, and sequentially washed in 70% ethanol and water before mounting it for photomicroscopy with an EOS Canon camera on a DMR1 Leica upright microscope equipped with 5 × and 16 × lenses. Enzymatically dissociated SAN myocytes were placed into chambers and allowed to attach to Cell-Tak-coated wells (3.5 μg cm −2 ) for 1 h (LAB-TEK II Chamber Slide, NUNC). Cells were then fixed with 4% paraformaldehyde for 20 min at RT, followed by soaking in 1 × PBS for several hours. Two hundred and fifty microlitres of 2% BSA (Sigma) containing mouse anti HCN4 monoclonal antibody (Neuromab, 1:100), rat anti HA monoclonal (Roche, 1:250) were added and allowed to incubate overnight at 4 °C in a humid chamber. Cells were rinsed for 4 × 15 min (1 × PBS). Goat anti-rat FITC secondary (Molecular Probes, 1:500), donkey anti mouse Alexa-647 (Molecular Probes, 1:500) and DAPI (4′,6-diamidino-2-phenylindole) were incubated for 90 min at RT followed by 4 × 15 min (1 × PBS). Prolong gold (Invitrogen) was overlayed and a glass coverslip gently placed over the sample. Images were taken with a Leica confocal microscope (Leica SPE). Image analysis was carried out on Metamorph Image Analysis software. Isolation of SAN, AVN and PF cells SAN and AVN myocytes were isolated from control and mutant mice, and individual PF cells were isolated from Mut/ Cx40 eGFP/+ mice as follows [31] , [32] : Hearts were removed under general anaesthesia using 10 mg kg −1 of xylazine (Rompun 2%, Bayer AG, Leverkusen, Germany) and 100 mg kg −1 of ketamine (Imalgène, Merial, Bourgelat, France). The SAN and AVN regions, as well as the endocardial ventricular tissue, were excised in pre-warmed (35 °C) Tyrode’s solution containing (in mM): NaCl 140, KCl 5.4, CaCl 2 1.8, MgCl 2 1, HEPES-NaOH 5 and D -glucose 5.5 (adjusted to pH 7.4 with NaOH). Tissue strips were then transferred into a ‘low-Ca 2+ -low-Mg 2+ ’ solution containing (in mM): NaCl 140, KCl 5.4, MgCl 2 0.5, CaCl 2 0.2, KH 2 PO 4 1.2, taurine 50, D -glucose 5.5, BSA, 1 mg ml −1 ; HEPES-NaOH 5 (adjusted to pH 6.9 with NaOH). Tissue was digested by Liberase TH (229 U ml −1 , Roche, Boulogne-Billancourt, France), elastase (1.9 U ml −1 , Boehringer, Mannheim, Germany) and 200 μM CaCl 2 . Digestion was carried out under manual mechanical agitation at 35 °C for 9–13 min. Tissue strips were then washed and transferred into a modified ‘Kraftbrühe’ medium containing (in mM): L -glutamic acid 70, KCl 20, KOH 80, (±) D -β-OH-butyric acid10, KH 2 PO 4 10, taurine 10, BSA 1 mg ml −1 and HEPES-KOH 10 (adjusted to pH 7.4 with KOH). Single SAN, AVN and PF cells were then isolated by agitation in Kraftbrühe solution at 35 °C. Cellular automaticity was restored by re-adapting the cells to a physiological extracellular Ca 2+ concentration by addition of a solution containing (in mM): NaCl 10, CaCl 2 1.8 and normal Tyrode’s solution containing BSA (1 mg ml −1 ). The final cell storage solution contained (mM): NaCl 100, KCl 35, CaCl 2 1.3, MgCl 2 0.7, L -glutamic acid 14, (±) D -β-OH-butyric acid 2, KH 2 PO 4 2, taurine 2, BSA 1 mg ml −1 (pH 7.4) and gentamycin (50 μg ml −1 ). All chemicals were from SIGMA (St Quentin Fallavier, France). Patch-clamp recordings of mouse SAN, AVN and PF cells The basal extracellular Tyrode’s solution used in all recordings contained (in mM): NaCl 140, KCl 5.4, CaCl 2 1.8, MgCl 2 1.0, HEPES-NaOH 5.0 and D -glucose 5.5 (adjusted to pH 7.4 with NaOH). Automaticity was recorded by the perforated patch-clamp technique using escin (30 μM); I f was recorded under standard whole-cell configuration. Patch-clamp electrodes had a resistance of 4–5 MΩ when filled with an intracellular solution containing (mM): K + -aspartate 130, NaCl 10.0, ATP-Na + salt 2.0, creatine phosphate 6.6, GTP-Mg 2+ 0.1, CaCl 2 0.04 (pCa 7.0) and HEPES-KOH 10.0 (adjusted to pH 7.2 with KOH). All experiments were carried out at 36 °C. All electrophysiological data were recorded and analysed using pCLAMP 9.2 (Molecular Devices, St Grégoire, France). All chemicals were from SIGMA (St Quentin Fallavier, France). Ca 2+ imaging and analysis of LCRs Spontaneous [Ca 2+ ] i transients and LCRs were recorded in SAN pacemaker myocytes loaded with Fluo-4 AM (20 μM, 35 min) at 36 °C. Images were obtained with confocal microscopy (Zeiss LSM 780) by scanning the myocyte with an Argon laser in line scan configuration (3.78 ms and/or 1.53 ms line rate); fluorescence was excited at 488 nm and emissions were collected at >505 nm. A × 63 oil immersion objective was used to record [Ca 2+ ] i in isolated SAN myocytes. Image analyses were performed by ImageJ software. Images were corrected for the background fluorescence and the fluorescence values (F) were normalized to the basal fluorescence (F0) to obtain the fluorescence ratio (F/F0). Integrals of light intensity were analysed by pCLAMP 9.2 (Molecular Devices). [Ca 2+ ] i parameters were analysed as follows: upstroke velocity of [Ca 2+ ] i transient was measured from the threshold to the peak of the [Ca 2+ ] i transient; [Ca 2+ ] i transient duration was measured from the threshold of [Ca 2+ ] i transients to 90% decay; and [Ca 2+ ] i transient recovery time was measured from the peak of the [Ca 2+ ] i transient to 90% decay. Image acquisition and analysis were performed on workstations of the Montpellier RIO Imaging facility. Measurements in isolated right atria The spontaneous beat frequency and its regulation in isolated atrial preparation from control and mutant mice were recorded in thermostated organ baths as described previously [64] . Effects of pharmacological activation of sympathetic function on HR response were examined by adding the adrenoceptor agonist ISO at cumulatively increasing concentrations (ISO, 0.001–1.0 μM). Effects of pharmacological blockade of I f were investigated by adding 0.3–1.0 μM IVA. Telemetric recordings of ECG and analysis For telemetric ECG recordings, adult male mice were anaesthetized with 2% isoflurane. A midline incision was made on the back along the spine to insert a telemetric transmitter (TA10EA-F20, Data Sciences International, ‘s-Hertogenbosch, The Netherland) into a subcutaneous pocket with paired wire electrodes placed over the thorax (chest bipolar ECG lead). Local anaesthesia was performed with lidocaine (1%) injected subcutaneously at the sites of electrodes and transmitter implantation. To manage possible post-surgery pain, Advil (paracetamol and ibuprofen, 7 ml l −1 ) was added to the drinking water for 4 days after implantation. Experiments were initiated at least 8 days after recovery from surgical implantation. Mice were housed in individual cages with ad libitum access to food and water, and were exposed to standard 12-h light–dark cycles in a thermostatically controlled room. ECG signals were recorded using a telemetry receiver and an analogue-to-digital conversion data acquisition system for display and analysis by Dataquest A.R.T. software. HRs were determined from interbeat (RR) intervals of the ECG. Mean HR values were obtained from each mouse for a 24-h period. For drug administration or exercise experiments, mean HR values were calculated in each mouse by analysing different periods of 5 min. ECG parameters were measured with ECG Auto 1.5.7 software (EMKA, Paris, France). Swimming tests were performed using customized Plexiglas boxes (15 × 32 × 13 cm (W × L × H)) filled with pre-warmed water (32 °C). Telemetric blood pressure recordings Mice with a body weight of >24 g were anaesthetized by intraperitoneal administration of ketamine/xylazine adapted to body weight. Telemetric transmitters (Physiotel PA-C10, Data Sciences International) were subcutaneously implanted with the sensing tip placed in the aorta via the left carotid artery. After 10 days of recovery from surgery, interventions and recordings (Dataquest A.R.T. software for acquisition and analysis) were started. For each mouse, blood pressure was continuously recorded for at least 48 h. For data analysis, mean blood pressure data were obtained for each consecutive minute within one recording period. The blood pressure mean data were then sorted by the corresponding activity in 7 bins between ‘0’ (no activity) and ‘7’ (activity >30 arbitrary units (aU)), and averaged over all mice. Data analysis Results are presented as means± s.e.m. Statistical significance was defined as P <0.05. Statistical tests used in each experiment are specified throughout the figure legends. Analysis was performed using Prism v6 (GraphPad Software). How to cite this article: Mesirca, P. et al . Cardiac arrhythmia induced by genetic silencing of ‘funny’ ( f ) channels is rescued by GIRK4 inactivation. Nat. Commun. 5:4664 doi: 10.1038/ncomms5664 (2014).